Imaging of molecular surface dynamics in brain slices using single-particle tracking Organization of signalling molecules in biological membranes is crucial for cellular communication. Many receptors, ion channels and cell adhesion molecules are associated with proteins important for their trafficking, surface localization or function. These complexes are embedded in a lipid environment of varying composition. Binding affinities and stoichiometry of such complexes were so far experimentally accessible only in isolated systems or monolayers of cell culture. Visualization of molecular dynamics within signalling complexes and their correlation to specialized membrane compartments demand high temporal and spatial resolution and has been difficult to demonstrate in complex tissue like brain slices. Here we demonstrate the feasibility of single-particle tracking (SPT) in organotypic brain slices to measure molecular dynamics of lipids and transmembrane proteins in correlation to synaptic membrane compartments. This method will provide important information about the dynamics and organization of surface molecules in the complex environment of neuronal networks within brain slices. Local organization and dynamics of transmembrane molecules are crucial parameters for cellular communication. Within small membrane compartments, as the neuronal synapse, the number of molecules is small, the availability of binding partners is limited and interactions might be biased by other competing binding partners, thereby influencing the establishment of long-lasting signalling complexes. Surface mobility of signalling molecules in the cell membrane contributes to the establishment, maintenance and modulation of signalling proteins within subcellular compartments as the neuronal synapse [1] , [2] . Whereas biochemical and molecular experiments often use isolated systems to control binding affinities and molecular composition of such complexes, a direct observation of the involved molecules and their interactions in the natural environment is missing. The lack of this information may lead to misinterpretations of signalling events under non-saturated conditions. For example, the formation and maintenance of adhesive contacts between T cells and antigen-presenting cells have been demonstrated to depend on the local mobility of binding partners, which strongly improves the speed of contact formation and maintenance [3] . In contrast, the stabilization of binding partners at saturating concentration of molecules could gain similar adhesive strength but could not compete for the speed of contact formation [4] . Within neuronal synapses, neurexins are presynaptic adhesion molecules important for synaptic transmission [5] . For inhibitory synapses, it has been suggested that the mobility of neurexins might be a mechanism for synapse formation and maintainance [6] . Hence, detailed information about temporal and spatial parameters like dwell-time and radius of confinement within a membrane compartment are important parameters to assess complex formation and affinity, but are difficult to obtain in complex cellular assemblies. One approach to sense such dynamic interactions are fluorescent recovery after photobleaching (FRAP) experiments. Here biological and technical limitations bias the recovery of the fluorescence and make it difficult to extract more information than an averaged recovery rate, interpreted as the mobile fraction of molecules. Also, the recycling of the surface pool of investigated molecules and the precision of the bleached membrane surface at different depths are weakly controlled. Therefore, any temporal or spatial improvement of the resolution will help to better understand the function of multimer signalling complexes and their dynamic organization. Recently, stimulated emission depletion microscopy has been used to localize synaptic molecules in living mouse brains [7] , [8] . Despite improved structural resolution, the temporal resolution remains low. In addition, stimulated emission depletion microscopy does not yet allow for the direct observation of individual molecules in such complex environments. Another method of investigation, which fullfills the temporal and spatial resolution requirements, is single-particle tracking (SPT) [9] . SPT comprises the detection of signals emitted from a defined light emitter, attached to the molecule of interest, the precise determination of its positions and the connection with the most likely position in the following time frame. Experimental constrains are the specificity of the labelling, the strength of the fluorescent signals and the labelling density, which has to be reasonably low so that extensive overlap of diffraction limited images of neighbouring fluorophores is avoided. The development of monomeric photoactivatable fluorescent proteins allows having stochastic activation of a small protein population at a given time point, described as photoactivation localization microscopy (PALM) [10] . Furthermore, it allows for having genetically encoded single-molecule specificity to label the protein of interest. This development makes PALM suitable for investigations of molecular surface organization of single molecules in living cells, leading to the development of sptPALM [11] . However, the application of sptPALM deep into complex environments, such as three-dimensional (3D) brain tissue, is strongly limited and requires complex instrumentation [12] , [13] . In particular, the axial resolution gained by relying on total internal reflection fluorescence microscopy or oblique illumination in monolayer cell cultures is lost within 3D brain tissue, which limits the application of sptPALM. Thus, labelling surface proteins via specific binding molecules like antibodies has several advantages. First, depending on the membrane turnover of the molecule of interest only the surface population of the molecule is detected and, second, the best suitable fluorophores for a particular environment can be selected. Finally, spatio-temporal dynamics of surface molecules can be investigated in the native cellular environment. Here we use quantum dots (QDs) as fluorescent probes. QDs are very stable fluorophores, their fluorescent quantum yield is >80%, their Stokes shift is exceptionally large and the surface of QDs can be functionalized for a large spectra of molecules [14] . Using a set-up including a fast confocal spinning disk unit (CSU), we are able to image QDs bound to cell-surface molecules in brain slices at depths up to 60 μm, which would not be accessible using conventional wide-field microscopes owing to light-scattering and the strong contribution of cellular autofluorescence. Optimized localization and monitoring of single-molecule mobility with high specificity was possible at depths up to 20 μm, having a subdiffraction-limited spatial localization accuracy of ~50 nm and a temporal resolution in the millisecond range. This approach enabled us to monitor molecular surface dynamics of membrane-associated molecules or transmembrane molecules within the complex environment of a cultured brain slice. Labelling and detection of single molecules in brain tissue Surface mobility of molecules is caused by the thermal motion of lipids within the lipid bilayer of membranes. We first monitored the mobility of the glycosylphosphatidylinositol (GPI)-anchored green fluorescent protein (GFP) in the outer leaflet of the plasma membrane of neurons and glial cells in brain slices that were labelled with anti-GFP QDs ( Fig. 1a–e , Supplementary Fig. 1d,e ). GPI–GFP has no direct interactions with intracellular scaffold proteins or extracellular binding partners and has been used to investigate lipid subdomains of the neuronal membrane, assuming only passive interactions [15] , [16] . The success of our SPT experiments in complex cellular environments relies on several factors: the specificity and accessibility of the label, the photo stability and brightness of the fluorophores as well as the optical accessibility and reliability of the fluorescent signal. 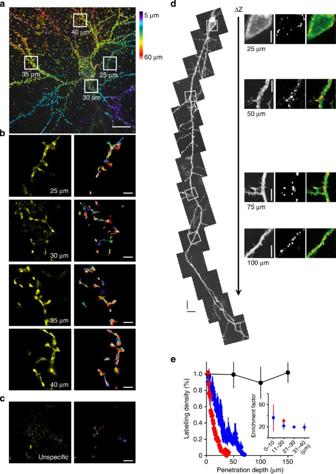Figure 1: SPT in organotypic brain slices using QDs coupled to a monoclonal antibody against GFP. (a) Z-projection of anti-GFP QDs inside an organotypic hippocampal slice acquired with our CSU set-up: anti-GFP QDs at dendrites of a GPI–GFP-transfected neuron were recorded at different depths inside the slice with an acquisition frequency of 10 Hz and an axial sampling rate of 0.1 μm. The colour encodes the z-depth of localized molecules within the stack projection, starting from 5 μm (blue) to 60 μm (deep red). Scale bar, 10 μm. (b) Magnified view of the positions of detected molecules at four different depths/locations, as indicated ina. Extracted trajectories are plotted with different colours in the right panel. Note that the labelling specificity remains similar between the four given examples. (c) Example of freely diffusing unspecific QDs. Note that the large cloud of detected QDs only results in very few trajectories because of the quick escape of QDs from the focal plane. Scale bar, 1 μm (b,c). (d) Projections of z-scans along a GPI–GFP-transfected neuron within an organotypic hippocampal slice using a two-photon microscope. Scale bar, 10 μm. Enlarged subregions at different depths show specific labelling with anti-GFP QDs without a loss of labelling density. Scale bar, 5 μm. (e) Quantification of relative labelling density for three experimental settings (red, single-photon excitation, oil immersion objective × 100/NA 1.4, blue, single-photon excitation, water immersion objective × 60/NA 1.1, black, two photon excitation, water immersion objective × 60/NA 1.1, error bars represent±s.e.m.). The labelling density was calculated by normalizing the number of QDs detected within optical slices to the density at 3 μm penetration depth. The inset demonstrates that there is only minor change in the specificity of labelling within the first 40 μm (error bars represent±s.e.m.). Data obtained with × 60/NA 1.1 water immersion objective are from 11 neurons in 7 organotypic slice cultures and data acquired with a × 100/NA 1.4 oil immersion objective are from 7 neurons in three slice cultures. Two-photon data are from six neurons in four slice cultures. Figure 1: SPT in organotypic brain slices using QDs coupled to a monoclonal antibody against GFP. ( a ) Z-projection of anti-GFP QDs inside an organotypic hippocampal slice acquired with our CSU set-up: anti-GFP QDs at dendrites of a GPI–GFP-transfected neuron were recorded at different depths inside the slice with an acquisition frequency of 10 Hz and an axial sampling rate of 0.1 μm. The colour encodes the z-depth of localized molecules within the stack projection, starting from 5 μm (blue) to 60 μm (deep red). Scale bar, 10 μm. ( b ) Magnified view of the positions of detected molecules at four different depths/locations, as indicated in a . Extracted trajectories are plotted with different colours in the right panel. Note that the labelling specificity remains similar between the four given examples. ( c ) Example of freely diffusing unspecific QDs. Note that the large cloud of detected QDs only results in very few trajectories because of the quick escape of QDs from the focal plane. Scale bar, 1 μm ( b , c ). ( d ) Projections of z-scans along a GPI–GFP-transfected neuron within an organotypic hippocampal slice using a two-photon microscope. Scale bar, 10 μm. Enlarged subregions at different depths show specific labelling with anti-GFP QDs without a loss of labelling density. Scale bar, 5 μm. ( e ) Quantification of relative labelling density for three experimental settings (red, single-photon excitation, oil immersion objective × 100/NA 1.4, blue, single-photon excitation, water immersion objective × 60/NA 1.1, black, two photon excitation, water immersion objective × 60/NA 1.1, error bars represent±s.e.m.). The labelling density was calculated by normalizing the number of QDs detected within optical slices to the density at 3 μm penetration depth. The inset demonstrates that there is only minor change in the specificity of labelling within the first 40 μm (error bars represent±s.e.m.). Data obtained with × 60/NA 1.1 water immersion objective are from 11 neurons in 7 organotypic slice cultures and data acquired with a × 100/NA 1.4 oil immersion objective are from 7 neurons in three slice cultures. Two-photon data are from six neurons in four slice cultures. Full size image First, we tested whether QDs are useable to access cells within cultured brain slices. We used polyethyleneglycol-coated QDs (605 nm), which have a reported size of about 30–35 nm (ref. 17 ), and detected their penetration by the use of a two-photon microscope. After 5 min incubation time, QDs were detectable throughout the entire tissue, proving that the penetration of QDs into cultured brain tissue is not a limiting factor. Next, we used brain slices transfected with GPI–GFP and incubated them with anti-GFP antibody-coated QDs. We observed specific labelling throughout the slice, covering transfected neurons and glia cells by using both, a spinning disc confocal as well as a two-photon microscope ( Fig. 1a–d , Supplementary Fig. 1a–d ). Here we observed two populations of QDs. One fraction specifically bound to the membrane of transfected cells ( Fig. 1a,b,d , Supplementary Figs 1a–d,2a , Supplementary Movie 1 ) and a second very mobile fraction of QDs with no specificity was freely diffusing within the extracellular space ( Fig. 1c ). The density of QDs on the membrane of transfected cells could be controlled by the concentration of QDs in the incubation media (usually we use 1–2 nM pre-coated QDs, see Methods section) and the time of incubation (usually 5 min). Increasing the incubation time up to 30 min resulted in higher labelling density but increased the risk to monitor intracellular uptake of QDs. We occasionally observed intracellular QDs, identified as QDs showing directed motion ( Supplementary Fig. 2b–d , Supplementary Movie 2 ). Transfected cells showed strong accumulation of QDs on the membrane up to 150 μm deep into the tissue ( Fig. 1d,e ), indicating that the penetration of QDs is not substantially hindered by adding the GFP antibody and that they do not loose specificity when penetrating into the tissue. This also indicates that the extracellular space (ECS) is much more permeable than suggested by ultrastructural investigations on fixed tissue [18] , [19] . Furthermore, it confirms in vivo measurements of the ECS in adult rat neocortex, described as fluid-filled ‘pores’ of about 38–64 nm using QDs as reporters [20] . To quantify QD mobility, we used an upright fluorescent microscope equipped with a × 60 water immersion objective, an Electron Multiplying Charge Coupled Device (EMCCD) camera and a CSU to gain confocal images at high acquisition rate within a large field of view. Owing to using one-photon excitation, the resulting light scattering and the refractive index mismatch degraded the localization accuracy and limited the detection of QDs to the first 60 μm of the brain tissue ( Fig. 1e ). In addition, brain tissue has often a prominent autofluorescence background, which renders the detection of single fluorophores difficult, especially if high temporal resolution is needed. We used QDs emitting between 605 and 655 nm because the autofluorescence of the neuronal tissue is reasonably low in this spectrum. The use of QDs with smaller core size, hence, smaller overall size and emission spectra <600 nm proved to be less suitable in these experiments because of the stronger autofluorescence of the tissue. Despite a high labelling specificity, the use of single fluorophore-tagged anti-GFP nanobodies in brain tissue was disadvantageous, particularly because of the weaker fluorescence signal compared with QDs ( Supplementary Fig. 3a ). QDs without polyethylene glycol coating are substantially smaller than coated ones [17] but caused strong unspecific labelling and were not further explored as an alternative to polyethylene glycol-coated QDs. Comparing the diffusion properties of QDs of different sizes (525–655 nm), corresponding to effective diameters of 25–45 nm [17] and anti-GFP nanobodies on GPI–GFP-transfected neurons in culture did not show major differences in the diffusion coefficient ( Supplementary Fig. 3e–g ). In fact, we observed rather an increase of immobile nanobody-tagged GPI–GFP molecules than an increase of mobile ones. Hence, we conclude that the probe size does not yield dramatic changes of the mobility of GFP-labelled GPI molecules in the neuronal membrane. Molecular dynamic within subcellular compartments The strong fluorescence of QD-labelled GPI–GFP molecules allowed monitoring the motion of these molecules at high acquisition rate (30 frames per second) with a lateral localization accuracy of ~100 nm, using a water immersion objective (Olympus × 60, 1.1 numerical aperture (NA)). Despite a sizeable drop of the signal-to-noise ratio (SNR) ( Supplementary Fig. 4 ), we could still detect QDs within the first 60 μm of the slice ( Fig. 1a–f , Supplementary Fig. S1a–d ). The localization accuracy of QDs strongly depends on the SNR [21] , which is depending on illumination power and acquisition speed. We adjusted the laser power between 50 and 400 mW, corresponding to 3–20 mW cm − 2 at the output of the objective, to find a compromise between the SNR and bleaching. The frame rate was kept at 30 Hz ( Supplementary Figs 2a,3 , Supplementary Movie 1 ). Using the water immersion objective and adjusting the correction collar of the objective, we could reduce the spherical aberrations induced by the refractive index mismatch. QD-labelled molecules were localized by a wavelet-based method performing well for data with low SNR described recently [22] and tracked over time using a simulated annealing algorithm [23] to quantify single-molecule dynamics [24] , [25] , [26] . We also tested the Gaussian fitting method for QD localization [27] , [28] and the Vogel algorithm for tracking individual QDs [29] , which yielded similar QD localization accuracy and dynamics but required much longer calculation times (the wavelet-based method worked 20 times faster with similar localization accuracy [22] ). The limitation of the localization accuracy, together with the limited trajectory lengths ( Fig. 2a ) deteriorated the precision of the diffusion coefficient. This was corrected by filtering out trajectories with less than 12 points. We computed linear fits of the mean square displacement (MSD) using the first eight points in slices in contrast to four points commonly used in primary cultures [30] . The stochastic blinking of QDs was not considered to connect neighbouring trajectory segments to avoid false connection of trajectory segments due to the 3D extension of neuron and glia cells in the tissue. About 40% of the localised QDs trajectories were ≥12 time points long. This proportion did not vary over penetration depth ( Fig. 2a,b ). Another effect of this filtering is the loss of short trajectories, which most probably represent either freely floating QDs in the extracellular space ( Fig. 1c ) or vertical moving QDs, escaping the focal plane. In primary cultures, trajectories were slightly longer, owing to the better SNR and the more planar cellular architecture. Diffusion properties of GPI–GFP expressed in slices were in the same order of magnitude as seen in dissociated hippocampal neurons and did not change with depth ( Fig. 2c ). Plotting MSD curves for QDs at different depths showed increasing confinement, illustrated in the stronger curvature of the MSD curve ( Fig. 2d ). Despite the possibility to sense lateral diffusion of molecules, the localization accuracy is not optimal to explore subcellular compartments such as synapses. Therefore, we configured our bath chamber in a way that we can introduce a coverslip between the objective and the slice culture, which allowed the use of oil immersion objectives with high NA ( Fig. 2e ). This clearly improved our localization accuracy (~50 nm, Fig. 2e,f ). Here organotypic slices are of great advantage. In contrast to acute slices where the first cell layers are often harmed by the slicing procedure, all cells are alive and integrated into the neuronal network after five to six days in vitro (DIV). Testing the viability of neurons close to the surface of the cultured slice by whole-cell patch-clamp recordings, we could confirm that normal electrical properties and spontaneous activity of neurons within the first cell layers of our slice cultures are preserved (5–21 DIV) ( Supplementary Table 1 ). Despite the stronger influence of the refractive index mismatch using the oil immersion objective, single QDs were clearly detectable within the first 20 μm ( Fig. 1e ). Again, we measured the surface mobility of GPI–GFP at axons, dendrites and synaptic compartments ( Fig. 3a–c ). The GFP fluorescence was used to identify neuronal compartments as dendrites, axons and cell soma. The postsynaptic location could be visualized by co-expression of the fluorescent marker Homer1C-DsRed. Within the example given in Fig. 3a , detected positions of anti-GFP QDs along transfected axons, dendrites and synaptic spines demonstrate different molecular mobility within the different membrane compartments ( Fig. 3a–e ). QDs detected outside transfected neurons were highly mobile and showed free Brownian motion as indicated by the MSD plot ( Fig. 3d,f ). The differences in the lateral dynamic of GPI–GFP between axonal, dendritic and synaptic membrane compartments were not different from the situation in primary cultures, as indicated by the overlap of the MSD plots and similar diffusion coefficients ( Fig. 3f–h ). Comparable results were reported previously in cultured hippocampal neurons [16] , [31] . Mobility differences between different compartments were due to a shift of the diffusive fraction without a significant change of the immobile fraction ( Fig. 3g ). Homer-DsRed-positive synapses were accessible for QDs bound to GPI–GFP molecules and showed frequent temporal confinement ( Fig. 3e ) similar to synaptic lipid mobility in cultured hippocampal neurons [16] , [31] . To describe the mobility of individual QDs over time within the synaptic compartment in more detail, we employed a method described by ref. 32 to detect temporal lateral confinement. An example is given in Fig. 3c,e showing the temporal confinement of QD-labelled GPI–GFP inside a spine head. Here confinement is defined as periods of time where a particle remains longer within a membrane area than predicted by assuming free Brownian diffusion. We analysed the population of molecules localized within the postsynaptic membrane or transiently passing the postsynaptic membrane. The analysis revealed that about 39.8±5.5% (mean±s.e.m., 2,085 trajectories within 250 synapses from 3 slice cultures) of the time within the synapse GPI–GFP molecules undergo temporal confinement. Molecules confined within Homer1C-positive clusters explored a membrane surface of about 0.18±0.12 μm in diameter (mean±s.e.m., 48 synapse, 3 slices), which is close to the size of a postsynaptic density, as described in quantitative electron microscopic studies [33] . Along the axon, GPI molecules diffused without strong confinement similar to free Brownian motion. The identical shape of the MSD curves while having differences in the absolute values ( Fig. 3f ) demonstrates that differences between neuronal membranes at various subcellular compartments are verifiable. It is also apparent that the diffusion in brain slices and cultured primary neurons is similar. To substantiate this conclusion, we overexpressed adhesion molecules at the pre- and postsynaptic side. The adhesion molecule neuroligin1–HA (Nlg1-HA) was expressed together with Homer1C–GFP. Nlg1-HA showed a lower mobility within the dendritic membrane compared with GPI–GFP ( Fig. 3j,k ). As described previously, the synaptogenetic effect of Nlg1 (ref. 34 ) could be observed by an increase in dendritic spine density and was taken as a confirmation for functional Nlg1-HA expression (spine density control 0.8±0.04 spines per μm (mean±s.e.m., n =16) versus spine density Nlg1-HA 1.5±0.1 spines per μm (mean±s.e.m., n =11)). Analysing trajectories of QD-labelled Nlg1-HA molecules that co-localized with Homer1C–GFP clusters, we found that the diffusion coefficient of mobile Nlg1-HA strongly decreased within postsynaptic spines, whereas the immobile population increased. Outside synapses, Nlg1-HA was significantly more mobile. During the time of observation (60 s), a fraction of Nlg1-HA molecules moved between synaptic locations, which is in agreement with the dynamic organization of Nlg1 within the postsynaptic membrane [35] . Since we did not see significant differences in the mobility of GPI–GFP molecules labelled with different QDs ( Supplementary Fig. 2 ), we co-expressed GPI–GFP and Nlg1-HA to confirm the difference in molecular mobility within the dendritic membrane. We labelled both molecules simultaneously, using QD605 and QD655 for the two tags -GFP and -HA. GPI–GFP QDs were much faster and less confined ( Fig. 3m,n ). Overexpression of β-neurexin–GFP, a prominent, mostly presynaptically expressed binding partner of Nlg1 (ref. 36 ), showed strong expression and high mobility at axons, which is in agreement with previous FRAP data obtained from inhibitory neurons in cultured slices [6] . 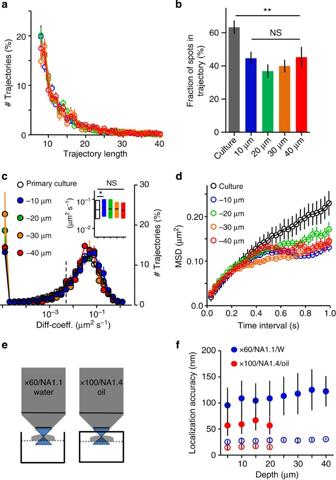Figure 2: Characterization of GPI–GFP mobility. (a) Distribution of trajectory lengths in different depths (minimal time points=8,n=33 neurons, 11 slice cultures). (b) The percentage of localizations that are included into trajectories ≥12 time points at different depths (data are represented as mean±s.e.m., differences tested by one-way analysis of variance followed by the Newman–Keuls multiple comparison test, **P<0.001). (c) Distribution of diffusion coefficients (D) of neuronal expressed GPI–GFP at different depth, the population withD<0.008 μm2s−1(dotted line) represents the immobile fraction (n=12,678 trajectories, 42 slices, 15 slice cultures). The inset shows mobile fraction (D>0.008 μm2s−1) with median and interquartile (IQR). Note there is no difference between different depths despite the difference between culture (white) and slices at 10 μm depth (blue). Differences were tested by the Kruskal–Wallis test followed by Dunn’s multiple comparison test (*P<0.05). (d) MSD shown for trajectories ≥34 time points at different depths. Data are same as inc. Note the similar initial slope but deviation in curvature of the MSD, indicating stronger confinement within slices (MSD of trajectories >29 time points, 42 slices, 15 slice cultures). (e) Sketch of experimental set-up for different objectives, dotted line indicates a nylon grid to allow medium perfusion during recording. The closed chamber was used for oil immersion objective. Slices within this chamber were imaged for ≤20 min. (f) Localization accuracy for different depths and different objectives at 30 Hz. Used laser powers are 400 and 100 mW for water immersion objective × 60/NA 1.1 and oil immersion objective × 100/NA 1.4, respectively. The oil immersion objective exhibits better localization accuracy but allows measurements within the first 20 μm only. Empty circles represent theoretical limit for the localization accuracy based on photon numbers21, filled circles denote localization accuracy computed from the s.d. of Gaussian fits to immobile QDs in living brain slices (see Methods: ‘Image analysis and statistics’). Data are represented as means±s.d., five slice cultures for the water, seven slice cultures for the oil objective. The number of QDs decreased as a function of depth and ranged from 51 to 12 and from 70 to 5 for water and oil objective, respectively. Figure 2: Characterization of GPI–GFP mobility. ( a ) Distribution of trajectory lengths in different depths (minimal time points=8, n =33 neurons, 11 slice cultures). ( b ) The percentage of localizations that are included into trajectories ≥12 time points at different depths (data are represented as mean±s.e.m., differences tested by one-way analysis of variance followed by the Newman–Keuls multiple comparison test, ** P <0.001). ( c ) Distribution of diffusion coefficients ( D ) of neuronal expressed GPI–GFP at different depth, the population with D <0.008 μm 2 s −1 (dotted line) represents the immobile fraction ( n =12,678 trajectories, 42 slices, 15 slice cultures). The inset shows mobile fraction ( D >0.008 μm 2 s −1 ) with median and interquartile (IQR). Note there is no difference between different depths despite the difference between culture (white) and slices at 10 μm depth (blue). Differences were tested by the Kruskal–Wallis test followed by Dunn’s multiple comparison test (* P <0.05). ( d ) MSD shown for trajectories ≥34 time points at different depths. Data are same as in c . Note the similar initial slope but deviation in curvature of the MSD, indicating stronger confinement within slices (MSD of trajectories >29 time points, 42 slices, 15 slice cultures). ( e ) Sketch of experimental set-up for different objectives, dotted line indicates a nylon grid to allow medium perfusion during recording. The closed chamber was used for oil immersion objective. Slices within this chamber were imaged for ≤20 min. ( f ) Localization accuracy for different depths and different objectives at 30 Hz. Used laser powers are 400 and 100 mW for water immersion objective × 60/NA 1.1 and oil immersion objective × 100/NA 1.4, respectively. The oil immersion objective exhibits better localization accuracy but allows measurements within the first 20 μm only. Empty circles represent theoretical limit for the localization accuracy based on photon numbers [21] , filled circles denote localization accuracy computed from the s.d. of Gaussian fits to immobile QDs in living brain slices (see Methods: ‘Image analysis and statistics’). Data are represented as means±s.d., five slice cultures for the water, seven slice cultures for the oil objective. The number of QDs decreased as a function of depth and ranged from 51 to 12 and from 70 to 5 for water and oil objective, respectively. 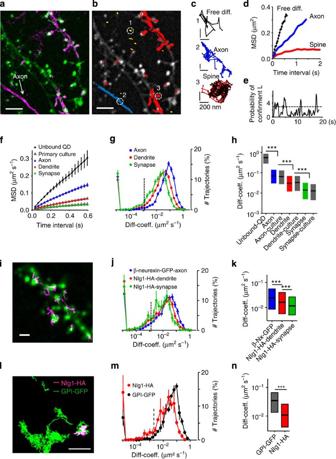Figure 3: QD dynamics in membrane compartments. (a) Image of dendrites expressing Homer1C-DsRed (green) and GPI–GFP (magenta). Positions of anti-GFP QDs, unspecific QDs are detected outside labelled neurits. (b) Individual trajectories of GPI molecules (red, dendrite; blue, axonal; yellow, extracellular), scale bar,10 μm (a,b). (c) Exemplary trajectories fromb: unbound QD (black), axonal (blue) and spine (red); scale bar, 200 nm. (d) MSD for trajectories inc. (e) Probability of confinement for spine trajectory, dotted line indicates level above which particles are considered to be confined. (f) MSD for unbound (black), axonal (blue), dendritic (red) and synaptic (green) trajectories, corresponding data from cultured neurons are similar (grey triangle). Data are means±s.e.m.,ntrajectories of >29 time points are included from 115 unbound QDs, 246/349 axonal slice/primary culture, 580/483 dendritic and 540/71 synaptic trajectories (72 slices (10 slice cultures), 10 cells (3 cultures)). (g) Distribution of diffusion coefficients (D) within subcellular compartments (axons, blue; dendrites, red; synapses, green). Data represented as mean±s.e.m., 21,390 trajectories, 72 slices, 10 slice cultures. (h) Mobile fraction of GPI–GFP within different subcellular compartments as median and IQR, differences between axons, dendrites and synapses were tested by the Kruskal–Wallis test followed by a Dunn’s multiple comparison test, ***P<0.0001, data are from 89 unbound QD, 2880/828 axon slice/culture, 7,690/994 dendrite and 2,425/282 synapse trajectories. (i) Dendritic segment, transfected with Homer1C–GFP (green) and trajectories of anti-HA-QD-labelled Nlg1-HA (magenta). (j) Distribution ofDof Nlg1-HA dendrites (red), synapses (green), β-neurexin–GFP axons (blue); error bars represent±s.e.m., data from 27 slices, 5 slice cultures. (k) Mobile fraction of Nlg1-HA and β-neurexin–GFP, median and IQR; differences were tested by the Kruskal–Wallis and Dunn’s multiple comparison test, ***P<0.0001, Nlg1-HA trajectories: 1,987 dendritic, 569 synaptic; β-neurexin trajectories: 2,529 axonal. (l) Exemplary trajectories of GPI–GFP (green) and Nlg1-HA (magenta) at co-transfected neuron, scale bars, 1 μm (i–l). (m) Distribution ofDfor Nlg1-HA (red) and GPI–GFP (black). (n) Mobile fraction of Nlg1-HA and GPI–GFP, median and IQR, data inmandninclude 607 trajectories for Nlg1-HA, 1,221 for GPI–GFP, 7 slices, 5 slice cultures; differences were tested by the Mann–Whitney test, ***P<0.0001. Full size image Figure 3: QD dynamics in membrane compartments. ( a ) Image of dendrites expressing Homer1C-DsRed (green) and GPI–GFP (magenta). Positions of anti-GFP QDs, unspecific QDs are detected outside labelled neurits. ( b ) Individual trajectories of GPI molecules (red, dendrite; blue, axonal; yellow, extracellular), scale bar,10 μm ( a , b ). ( c ) Exemplary trajectories from b : unbound QD (black), axonal (blue) and spine (red); scale bar, 200 nm. ( d ) MSD for trajectories in c . ( e ) Probability of confinement for spine trajectory, dotted line indicates level above which particles are considered to be confined. ( f ) MSD for unbound (black), axonal (blue), dendritic (red) and synaptic (green) trajectories, corresponding data from cultured neurons are similar (grey triangle). Data are means±s.e.m., n trajectories of >29 time points are included from 115 unbound QDs, 246/349 axonal slice/primary culture, 580/483 dendritic and 540/71 synaptic trajectories (72 slices (10 slice cultures), 10 cells (3 cultures)). ( g ) Distribution of diffusion coefficients ( D ) within subcellular compartments (axons, blue; dendrites, red; synapses, green). Data represented as mean±s.e.m., 21,390 trajectories, 72 slices, 10 slice cultures. ( h ) Mobile fraction of GPI–GFP within different subcellular compartments as median and IQR, differences between axons, dendrites and synapses were tested by the Kruskal–Wallis test followed by a Dunn’s multiple comparison test, *** P <0.0001, data are from 89 unbound QD, 2880/828 axon slice/culture, 7,690/994 dendrite and 2,425/282 synapse trajectories. ( i ) Dendritic segment, transfected with Homer1C–GFP (green) and trajectories of anti-HA-QD-labelled Nlg1-HA (magenta). ( j ) Distribution of D of Nlg1-HA dendrites (red), synapses (green), β-neurexin–GFP axons (blue); error bars represent±s.e.m., data from 27 slices, 5 slice cultures. ( k ) Mobile fraction of Nlg1-HA and β-neurexin–GFP, median and IQR; differences were tested by the Kruskal–Wallis and Dunn’s multiple comparison test, *** P <0.0001, Nlg1-HA trajectories: 1,987 dendritic, 569 synaptic; β-neurexin trajectories: 2,529 axonal. ( l ) Exemplary trajectories of GPI–GFP (green) and Nlg1-HA (magenta) at co-transfected neuron, scale bars, 1 μm ( i – l ). ( m ) Distribution of D for Nlg1-HA (red) and GPI–GFP (black). ( n ) Mobile fraction of Nlg1-HA and GPI–GFP, median and IQR, data in m and n include 607 trajectories for Nlg1-HA, 1,221 for GPI–GFP, 7 slices, 5 slice cultures; differences were tested by the Mann–Whitney test, *** P <0.0001. Full size image We present the application of SPT to cultured hippocampal brain slices, which are widely used as a model to combine acute genetic/molecular manipulation with physiological read-outs for neuronal plasticity. This new application allows for verification of interactions found in biochemical or molecular biology experiments in primary neuronal cultures, and will help to gain more detailed information about molecular organization and dynamics in complex tissue. In contrast to FRAP experiments, SPT allows to monitor diverging diffusion behaviours of individual proteins during neuronal activity within physiologically relevant time periods (msec to min). Observation of large populations of molecules with high temporal and spatial resolution will provide sufficient detail to significantly quantify effects on subpopulations of membrane-associated molecules. The accuracy with which the molecular dynamics can be described is mainly constrained by the optical accessibility of the tissue, which limits the application of SPT to the first cell layers in our system. Despite this limitation, the surface mobility of GPI–GFP molecules was determined to be comparable to the situation in primary cell cultures ( Figs 2 and 3 ). Nevertheless, as indicated by the stronger curvature of the MSD, we assume that the surface mobility might be restricted within the complex environment of the brain slice ( Fig. 2d ). However, despite this stronger confinement, the extracellular space is large enough for penetration of anti-GFP QDs throughout the slice within a few minutes ( Fig. 1d,e , here we monitored up to 150 μm). Also, it allows for diffusion of QDs between neighbouring cells as also monitored in intact rat brain [20] . Apparently, the ECS is much less packed as interpreted from electron microscopy-based analysis of fixed samples [18] . Whether the stronger confinement of QDs is caused by their size or potential polyvalence could not be proven directly, since the fluorescent signal of labelled nanobodies is too weak to be detected within slices in our set-up. In primary neuronal cell cultures, we could detect nanobody-labelled individual GPI–GFP molecules. The diffusion coefficient of the mobile fraction of QD-labelled GPI–GFP was slight but significantly higher than for the mobile fraction of monovalent nanobodies ( Supplementary Fig. 3g ), accompanied by an increased fraction of immobile nanobodies. These differences between nanobodies and QDs might result from a more efficient labelling of molecules in spatially restricted environments as synapses or cellular contacts to the coverslip, but point against a major impact of the QD on the lateral mobility of GPI–GFP molecules in the membrane. Previously, it has been observed that the use of smaller probes than antibody plus QD lead to a substantial increase in the number of detectable molecules without affecting the diffusion coefficient [27] . The SNR of very bright QDs is sufficient to monitor molecular dynamics within thick neuronal tissue and allows for detection of a diffusive range that is large enough to monitor differences in the mobility at different subcellular compartments ( Fig. 3a–e ). Furthermore, based on the wide excitation spectrum and narrow emission spectra of QDs, several molecules can be observed simultaneously ( Fig. 3l–n ). New molecular tools to label side-specific trans synaptic-interacting molecules promise to be useful to study the dynamic of, for example, adhesive contacts of the here separately monitored binding partners Nlg1-HA and β-neurexin–GFP [37] . In addition, the occasionally observed intracellular transport of endocytosed QDs into neurons opens the possibility to monitor processes like intracellular vesicle transport within brain slices. In fact, the lack of equivalent data for molecular dynamic in living tissue has led to the assumption that owing to manifold structures that might influence the stability of synaptic contacts [38] the mobility at synaptic contacts is much more restricted in brain slices. Thus, application of molecular imaging techniques in complex environments like brain slices will allow us to assess the impact of molecular dynamic on the local density of signalling molecules in small membrane compartments like the synapse. Using PALM, it was shown that the density of the inhibitory scaffold protein gephyrin is lower in synapses of cultured spinal cord neurons than in synapses from fixed spinal cord slices [39] . This indicates that the molecular organization and dynamic depend on the local cellular environment. The use of a well-established and affordable set-up makes our technique accessible for many researchers. In addition, our method will allow for the combination of SPT techniques with standard electrophysiological methods to probe how local rapid changes in molecular organization/density affect neuronal communication, as suggested for the incorporation of extrasynaptic AMPARs in the synapse after induction of long term potentiation (LTP) [40] , [41] . Combining with faster two-photon imaging would extend the application of SPT to deeper cell populations ( Fig. 1d,e ). It might open the possibility to perform SPT in acute brain slices by using specific antibodies to endogenous membrane proteins or knock-in mouse models. Hippocampal cell culture and organotypic slice culture Primary hippocampal cultures were prepared from embryonic wistar rats day 18 as described in ref. 42 . Briefly, cell suspensions obtained after dissociation with trypsin were plated onto poly- L -lysine (Sigma)-coated 18 mm glass coverslips (Menzel-Glaeser, Braunschweig, Germany) at a density of 20,000 cells per coverslip. After 1–2 h in MEM plus horse serum at 37 °C, five coverslips were transferred into a 35-mm dish containing a 70–80% confluent monolayer of astrocytes in neurobasal medium supplemented with B27 and 5 mM glutamine. Cultures were maintained at 37 °C in a humidified incubator with an atmosphere of 95% air and 5% CO 2 . Neurons were transfected at DIV 4 using Effectene transfection reagent (Qiagen) according to the manufacturer’s protocol. Experiments were performed between DIV 14 and 21. Organotypic slice cultures were prepared as described in ref. 43 with minor modifications. Briefly, using a McIllwain tissue chopper, 350 μm thick hippocampal slices were obtained from postnatal day 4–6 Bl6 wild-type mice and cultured on MillicellCell Culture Inserts (Millipore, 0.4 μm, Ø 30 mm) at 37 °C/5% CO 2 in culture medium composed of 50% Neurobasal medium, 25% Hank’s balanced salt solution (without MgCl 2 /without CaCl 2 ) and 25% horse serum supplemented with B27 (GIBCO, Invitrogen), 200 mM L -glutamine and 0.65% D (+)glucose (medium without phenol red). On the day of dissection, slices were transfected using a hand-held Helios gene gun (Bio-Rad). The plasmid DNA was coupled to gold microcarriers (1.6 μm diameter, Bio-Rad) by precipitation with calcium chloride according to the Bio-Rad’s Instruction Manual. Briefly, 7 μg gold microcarriers were resuspended in 100 μl ultra-pure water and mixed with 1–10 μg DNA and 40 μl spermidine (250 mM). This emulsion was filled up with water to a volume of 200 μl and precipitated with 200 μl CaCl 2 (1 M). After three times washing with dry 100% ethanol (Merck) and short sonication, the pellet containing the DNA-bound microcarriers was resuspended in 3.5 ml ethanol and enriched with 0.5 ml polyvinylpyrrolidone (0.05 mg ml −1 ) to help coating of the microcarriers to the inner wall of the teflon tubing (Bio-Rad). After loading and settling of the emulsion, the tubing was dried with nitrogen for 5 min and cut into little cartridges. Finally, the cartridges were put into the revolver of the gene gun and the microcarriers were shot from the cartridges onto the target tissue with helium pulse. Slices were fed twice a week by replacing half of the medium and imaged between DIV5 and DIV21. Cartridges were stored in parafilm-sealed 50 ml falcon tubes at 4 °C for up to 4 months. Plasmids and antibodies Plasmids were kindly provided by our collaborators: pCMV–GFP–GPI and pCMV–HA-Nlg1 (Olivier Thoumine, Bordeaux/Peter Scheiffele, Basel), pCMV–Homer–GFP (Daniel Choquet, Bordeaux), pSyn5-HA-neurexin1ß (Markus Missler, Münster). Primary antibodies used were the following: anti-GFP mouse IgG, monoclonal antibody (200 μg; clones 7.1 and 13.1; Catalogue number 11814460001; Roche Diagnostics) and anti-HA high affinity, rat monoclonal antibody (clone 3F10; 50 μg; Catalogue number 11867423001; Roche Diagnostics), anti-GFP nanobodies ATTO488 (Chromotek). Secondary antibodies used were the following: Qdot655 goat F(ab′) 2 anti-mouse IgG conjugate (H+L) (1 μM solution Q11022MP Lot729518; Invitrogen/Molecular Probes). For dual colour imaging the following were used: Qdot605 goat F(ab')2 anti-mouse IgG conjugate (H+L) (1 μM solution, Q11002MP; Invitrogen/Molecular Probes) plus Qdot655 goat F(ab')2 anti-rat IgG conjugate (H+L)(1 μM solution, Q11621MP; Invitrogen/Molecular Probes). Coupling of QDs to antibodies and slice incubation PBS (7.0–7.5 μl) were mixed in a microtube with 0.5–1.0 μl primary antibody and 1 μl QDs, and vortexed for 5 min at low speed (total volume 9 μl). Subsequently, 1 μl of casein (10 × Casein Solution, Vector Laboratories Inc; Burlingame, CA, 94010) was added to the tube and vortexed for an additional 5 min. A 35-mm Petri dish was covered with parafilm and a drop of 100 μl conditioned medium was added. The antibody-coupled QDs were added at a dilution of 1:1,000 (so 1 μl of the above-prepared solution) and mixed. Then, using a scalpel a slice was cut out from the membrane and transferred to the drop in the Petri dish. The Petri dish was returned to the incubator for 5–10 min. After, the slice was washed three times in HEPES-buffered extracelluar solution containing 0.5-1% BSA (albumin from bovine serum; Sigma A7638 10 G). For imaging, slices were transferred in HEPES-buffered extracellular solution (containing in mM: 145 NaCl, 2.5 KCl, 2 MgCl 2 , 2 CaCl 2 , 10 HEPES and 10 D -glucose, pH 7.4). Evaluation of the labelling specificity We expressed enhanced GFP-glycophosphatidylinositol (GFP–GPI) in neurons of cultured brain slices extending their QD-labelled neurites deeply into the tissue with high epitope specificity. The labelling specificity of QDs coupled to primary antibodies was determined by counting QDs on transfected neurons versus QDs in the background volume at different axial positions of 3D optical stacks using Imaris software (Bitplane AG, Zurich, Switzerland). Stacks were processed by 3D-blind deconvolution algorithm implemented in Auto Deblur X2 software (Media Cybernetics) with 10 iterations. Resulting image stacks were normalized by a linear histogram stretching and 3D rendered using Imaris. The Imaris spot detection wizard (sphere detection: × 60: x , y =1 μm; z =1 μm and for × 100: x , y =1 μm; z =3 μm) was used to segment and count all QDs based on the same threshold for all images. Segmentation of specific labelling was performed using the surface wizard of Imaris 7, which generates surfaces according to an intensity-based threshold. We further evaluated an enrichment factor by counting QDs on specific structures versus the background (both normalized to the respective specific or unspecific volume). Single-particle tracking Time-lapse recordings of QD-labelled molecules were acquired at 33–35 °C in a perfusion chamber mounted onto an upright microscope (Olympus BX50, Olympus, Japan) equipped with a spinning disk (CSU X1, Yokogawa, Japan) and × 60, 1.1 NA water immersion or × 100, 1.4 NA oil immersion objective. Images were acquired with a back-illuminated thinned EMCCD camera (iXon 897Andor, 512 × 512 pixels, pixel size 16 × 16 μm 2 ). QDs were excited by a 488-nm laser, tuneable between 0 and 1,000 mW. Fluorescence emission was collected through filters HQ605/40 and 655WB40. Time-lapse recordings of QDs were obtained with an integration time of 10–30 ms with up to 2,000 consecutive frames using Andor IQ software. QD-labelled molecules were tracked on randomly selected dendritic and axonal regions. Z-stacks, cellular structures and synaptic markers were acquired before and after QD recording. Two-photon imaging of QD tissue penetration The custom-built two-photon imaging set-up was based on an Olympus BX51WI microscope equipped with a LUMPlan W-IR2 60 × 0.9 NA objective. The hardware was controlled by ScanImage [44] written in Matlab. An ultrafast, tunableTi:Sapphire laser (MaiTaiDeepSee, Spectra-Physics) controlled by an electro-optic modulator (350-80, Conoptics) was used to excite QDs at 980 nm. Fluorescence was collected through the objective and the oil immersion condenser (1.4 NA, Olympus) with two pairs of photomultiplier tubes (H7422P-40, Hamamatsu). In both light paths, 560 DXCR dichroic mirrors and 525/50 and 607/70 emission filters (Chroma Technology) were used to separate green and red fluorescence. Infrared excitation light was blocked by short-pass filters (ET700SP-2P, Chroma Technology). Slice cultures were imaged after a 5-min incubation period with a Qdot655-conjugate as described above. Pixel image (512 × 512) frames (32 × 32 μm 2 ) were acquired at 0.5 μm increments between 0 and 200 μm starting at the surface of the slice culture. Frames (3 × 150; 30 Hz) were acquired per section and average number of QDots per frame was extracted for each section. Image analysis and statistics Localization of single QDs was performed using two-dimensional Gaussian fitting [27] or wavelet-based algorithm [22] . Single QDs could be identified by their blinking signature and their diffraction-limited size. The trajectories of QDs bound via an anti-GFP or anti-HA antibody to GFP- and HA-tagged molecules were reconstructed by simulated annealing algorithm [23] , taking into account molecule localization and total intensity. The blinking properties of QDs did not allow the recording of trajectories as a continuum. To avoid mis-reconnections between trajectories, sub-trajectories of the same QDs were analysed as individual trajectories. The dynamic behaviour of single molecules was computed from the MSD curves for all trajectories of at least 12 frames. Diffusion coefficients were calculated by linear fit of the first eight points of the MSD plots on dendrites, spines and axons. The resolution limit for diffusion coefficient obtained from trajectories acquired with the × 100, 1.4 NA oil immersion objective was 0.002 μm 2 s −1 obtained from recordings of fixed QDs within 10–20 μm range. The confinement index and explored surface were calculated according to refs 32 , 45 using custom software as described in ref. 46 . In brief, synaptic trajectories (Homer1C-positive membrane areas) were examined to identify periods of confined diffusion using the L function [32] . The confinement is defined by the instant diffusion coefficient of a molecule and the explored surface within a time period. A molecule is considered as confined if it remains in a region of radius R longer than expected by Brownian diffusion. The probability that a molecule remains confined within that region was calculated for trajectories localized in synaptic compartments. Each point of the trajectory was used as a starting point to calculate the instant diffusion coefficient and the probability of confinement [46] . To determine the area of confinement, exponential functions were fitted to the MSD( t ) plot for detected periods of confinement. The localization accuracy of our data was provided from two different methods. First, based on the number of photons, the background noise and the sampling, we computed the theoretical limit of the localization accuracy [21] , equation (17), and second, by computation of the s.d. of the localization coordinates obtained from repeated measurements of immobile QDs. Localization accuracy in living tissue were selected from immobile QDs, identified by their flat MSD curve over time. QDs dried under the coverslip were used in Supplementary Fig. 4c–f . The two methods for localization accuracy estimation exhibit similar courses of the curve but differ in their absolute values. The theoretical estimation yields much better accuracy than the estimation involving localized QDs. This is reasonable as the theoretical estimation computes the lower bound for the best localization accuracy that can be achieved by acquisition of a certain number of photons. In contrast, extraction from the s.d. of Gaussian fits computes the average accuracy and considers further important factors that influence the experimental localization accuracy. In particular, optical aberrations introduced by the refractive index mismatch and the long-distance observation, together with the thermal drifts of the microscope are source of localization estimation errors. In addition, the selection of truly immobile QDs in living tissue from flat MSD is difficult, since this is also the signature of highly confined molecules. The SNR is computed by ( I 0 − I b )/ σ . Here I 0 − I b designates the mean intensity above the background of a QD, computed from all pixels within its full width at half maximum. The variable σ denotes the noise of the objects’ signal, which is estimated from the residuals of the Gaussian fitting on the QDs’ intensity profile. Electrophysiology Neurons in hippocampal organotypic cultures were functionally characterized by the use of the whole-cell patch clamp technique. Patch pipettes were pulled from borosilicate glass and had resistances between 3 and 5 MΩ when filled with (mM): 145 potassium gluconate, 2 MgCl 2 , 10 HEPES, 0.1 EGTA, 2 Mg-ATP, 0.3 Na-GTP (pH 7.4 with KOH). The bath artificial cerebrospinal fluid contained (mM): 124 NaCl, 4.9 KCl, 2 MgSO 4 × 7 H 2 O, 2 CaCl 2 × 2 H 2 O, 1.2 KH 2 PO 4 , 25.6 NaHCO 3 , 20 glucose (pH 7.4, carbogen buffered). Currents were recorded with an EPC 9 amplifier (HEKA Electronics, Lambrecht Germany) controlled by Patchmaster software (HEKA Electronics). Spontaneous excitatory postsynaptic currents were recorded in whole-cell voltage clamp mode with a series resistance <15 MΩ. Action potential properties as amplitude, half width and threshold as well as resting membrane potential were recorded in the current-clamp mode without application of a holding current. Liquid junction potential of 10 mV was not subtracted from the data. Data were analysed by the use of the Fitmaster software (HEKA Electronics) and mini-analysis (Synaptosoft, USA). Influence of the laser power on the localization properties Localization accuracy can be easily improved by increasing the laser excitation power until a saturation plateau is reached. Here we employed a tuneable laser (488 nm, Genesis, Coherent), providing up to 1,000 mW output power. Because of the fibre coupling (Schäfter, Kirchhoff, Hamburg, Germany) and the transition through the CSU, the resulting excitation power between the CSU and the objective was only about 8% of the output laser power (see Supplementary Fig. S3b ). The resulting excitation power at the focal plane of the different objectives was about 5% and 3% of the output laser power for the × 60 water and × 100 oil objective, respectively. As immersion medium, we used purified water for the × 60 water and Zeiss Immersol 518 F for the × 100 oil objective. The rear apertures of both objectives are big enough to receive the complete laser beam from the CSU. However, the aperture of the microlenses of the CSU is fixed and cannot be adjusted to the individual objectives. To analyse the influence of laser power on the key detection performance parameters of our set-up, we imaged immobilized QDs (655 nm emission wavelength) that were dried under a coverslip (see Supplementary Fig. S4c,d ). This also gives us realistic best bounds for the performance of our set-up. Clearly, the localization accuracy improves with increasing excitation power and for the water objective prominent saturation starts after 400 mW. The oil objective showed no clear point of saturation. Changes in laser power are most efficient in the range of 100–400 mW, and as a compromise between detection performance and bleaching we choose 400 mW for experiments with the water objective and 100 mW for the oil objective. We also computed the dependency of the acquisition frame rate on the localization accuracy ( Supplementary Fig. S4e,f ) at optimal excitation laser power. Advantages of confocal spinning disk set-ups The main principle of a CSU is the creation of parallel laser beams, each working like a single confocal microscope. The laser beam is spread on a rotating disk equipped with microlenses that focus several parallel beams through the pinholes of the Nipkow disk. Each beam is focused on the specimen, exciting only a discrete spot. Emitted light passes the pinholes again and is collected on an EMCCD camera chip. By rotation of the disks, our CSU creates a full image every 30°. Confocal spinning disk microscopes basically parallelize confocal scanning, thus allowing very high frame rates. A disadvantage is the loss of illumination intensity due to the disks despite the use of microlenses, which we further compensate by increasing the laser power. Wide-field microscopes illuminate the whole field of view. This yields a decrease of the image contrast due to out-of-focus emitted light from the tissue above and below the focal plane. Their larger depth of field prohibits their use in the case of imaging thick living tissue. How to cite this article: Biermann, B. et al . Imaging of molecular surface dynamic in brain slices using single-particle tracking. Nat. Commun. 5:3024 doi: 10.1038/ncomms4024 (2014).